Structural mechanism of ergosterol regulation by fungal sterol transcription factor Upc2 Transcriptional regulation of ergosterol biosynthesis in fungi is crucial for sterol homeostasis and for resistance to azole drugs. In Saccharomyces cerevisiae , the Upc2 transcription factor activates the expression of related genes in response to sterol depletion by poorly understood mechanisms. We have determined the structure of the C-terminal domain (CTD) of Upc2, which displays a novel α-helical fold with a deep hydrophobic pocket. We discovered that the conserved CTD is a ligand-binding domain and senses the ergosterol level in the cell. Ergosterol binding represses its transcription activity, while dissociation of the ligand leads to relocalization of Upc2 from cytosol to nucleus for transcriptional activation. The C-terminal activation loop is essential for ligand binding and for transcriptional regulation. Our findings highlight that Upc2 represents a novel class of fungal zinc cluster transcription factors, which can serve as a target for the developments of antifungal therapeutics. Ergosterol is the major fungal membrane sterol that regulates membrane fluidity, plasma membrane biogenesis and function [1] . Ergosterol homeostasis is critical for fungal cells. Part of this regulation involves the transcription control of genes encoding ergosterol biosynthetic enzymes and proteins that perform sterol processing and uptake [2] . In some fungal species, such as Schizosaccharomyces pombe , it is mediated by hypoxic regulatory proteins, Sre1 and Scp1, which share common features with the mammalian sterol regulatory element-binding proteins (SREBPs) and SREBP cleavage-activating protein [3] , [4] . However, many other fungal species, including Saccharomyces cerevisiae and Candida species, lack protein homologues of the mammalian cholesterol regulators and appear to have evolved distinct regulatory mechanism [5] . In S. cerevisiae , Upc2 and Ecm22, two similar zinc finger transcriptional factors, have been implicated in ergosterol regulation by binding to the promoters of ergosterol biosynthetic and sterol uptake genes and activating the transcription on sterol depletion [2] , [6] . In addition, S. cerevisiae Upc2 is important for adaptation to hypoxia regulating up to one-third of anaerobically expressed genes [7] . Upc2 contains an amino-terminal (N-terminal) DNA-binding domain characterized by a conserved Zn(II) 2 -Cys 6 zinc finger motif and a carboxyl-terminal (C-terminal) conserved domain of unknown function. Owing to the essential role of ergosterol in fungal membranes, azole drugs that inhibit ergosterol biosynthesis are widely used for the treatment of fungal infections. Candida albicans is responsible for a large proportion of infections in immunocompromised individuals and the emergence of drug-resistant strains is of medical concern [8] . Resistance to azole drugs is partly due to the alteration of the ergosterol biosynthetic pathway. Many gain-of-function mutations in Upc2 that contribute to the drug resistance were identified in clinical isolates [8] . Mutations in the C-terminal domain (CTD) of Upc2 (A643V, A643T or G648D in C. albicans Upc2) result in the constitutive activation of the transcription factor (TF), resulting in the upregulation of ergosterol synthesis pathway and sterol uptake, which leads to a decreased susceptibility of the strains to azole drugs [9] , [10] . The gain-of-function mutation, G888D, in S. cerevisiae Upc2 results in the constitutive activation of the TF with a high level of aerobic sterol uptake [11] , [12] . These constitutive activation mutations are in close proximity in the C-terminal portion of Upc2, which may indicate that the CTD is important for the regulation of its transcriptional activity [9] . The CTDs of Upc2 and Ecm22 have no recognizable similarities to any characterized protein domains of known structures. However, conservation of this region across a large number of zinc TFs in many fungal species indicates that the CTD may represent a novel domain [13] . Deletion of UPC2 in pathogenic fungi, C. albicans and C. glabrata , leads to a significant decrease of tolerance to azole drugs and deletion of both UPC2 and ECM22 in S. cerevisiae is lethal in certain yeast strains [6] , [14] , [15] . Therefore, the Upc2 pathway may represent a potential co-therapeutic target for enhancing azole activity against these organisms [16] . Nuclear receptors (NRs) are soluble proteins that can bind to specific DNA-regulatory elements and acts as promotor-specific regulators of transcription. The activity of most NRs is modulated by binding of small lipophilic molecules [17] . Recent studies proposed that several members of the fungal zinc cluster family of transcription regulators may represent functional analogues of metazoan NRs [13] . Transcriptional activity of Oaf1/Pip2 is regulated by oleate binding to the CTD with similar ligand-binding characteristics and coactivator requirements to mammalian PPAR/RXR receptors [18] , [19] . Pdr1 zinc TFs bind to diverse xenobiotics and stimulate expression of drug efflux pumps resulting in induction of multidrug resistance in S. cerevisiae and C. glabrata , which is functionally similar to the regulation of multidrug resistance in vertebrates by the PXR NR [19] , [20] . However, due to the lack of structural and biochemical information of the fungal zinc finger transcriptional factors, the characteristics of this gene family have remained elusive. In this study, we have determined the crystal structure of the CTD of Upc2 from S. cerevisiae . We discovered that the CTD of Upc2 is a ligand-binding domain (LBD) for fungal sterols that regulate the transcriptional activity and cellular localization of Upc2 in a ligand-dependent manner. Upc2 displays conceptual similarities in domain architectures and the regulation of transcription activity to mammalian NRs. However, Upc2 LBD displays a distinct structural fold compared with the LBDs of metazoan NRs suggesting that Upc2 represents a novel class of zinc finger TFs. This study reveals that fungal zinc cluster TFs might be suitable targets for the developments of small drugs that could aid current antifungal therapy. Upc2 is a specific receptor for ergosterol Upc2 and Ecm22 share a high level of sequence similarity in the N-terminal DNA-binding domains characterized by a conserved Zn(II) 2 -Cys 6 zinc finger motif [21] . The C-terminal conserved region of about 300 amino-acid residues contains a transcription activation domain ( Fig. 1a ). Since the transcriptional activity of Upc2 is dependent on ergosterol levels in the cell, we hypothesized that the CTD may serve as a LBD for ergosterol and regulate transcriptional activity of Upc2. Dehydroergosterol (DHE) is a natural sterol with intrinsic fluorescence properties, which is found in low amounts in S. cerevisiae [22] , [23] . DHE is very similar to ergosterol in structural and chemical properties with only single double bond difference and it can replace ergosterol in yeast without any functional interference [24] . To test whether Upc2 directly binds to yeast sterols, we performed the fluorescent DHE-binding assay using purified CTDs of recombinant Upc2 (residues 598–913). Tryptophan residues of Upc2 were excited at 285 nm and the fluorescence spectrum of DHE was monitored. Spectral analysis revealed that tryptophan quenching at 340 nm was concomitant with the appearance of three emission peaks at 354, 373 and 393 nm ( Fig. 1b ). These peaks are characteristic of DHE, which suggests fluorescence resonance energy transfer (FRET) from Upc2 LBD to bound DHE [25] , [26] . Upc2 LBD binds free DHE with nanomolar affinity as measured by equilibrium-binding experiments ( Fig. 1b ). Upc2 LBD also extracts and binds DHE embedded in the DOPC (1,2-dioleoyl- sn -glycero-3-phosphocholine) liposomes as monitored by the increase of fluorescence emission at 375 nm when Upc2 LBD was added to DOPC:DHE liposomes ( Fig. 1c,d ). When non-fluorescent ergosterol was added to the mixture containing DHE-bound Upc2, the fluorescence emission was decreased indicating that ergosterol competes with DHE for the binding to Upc2. However, the addition of cholesterol did not affect the DHE binding indicating that Upc2 does not bind cholesterol. Other sterols such as 20-hydroxycholesterol, 25-hydroxycholesterol, hydrocortisone and β-estradiol did not compete with DHE suggesting that Upc2 LBD is a specific receptor for fungal sterols such as ergosterol and DHE ( Fig. 1e ). In addition, to examine the DHE and ergosterol extraction properties of Upc2 from the liposomes with a physiological lipid composition of yeast plasma membranes [27] , we monitored the extraction of DHE from the liposomes with phosphatidylcholine/phosphatidylethanolamine/phosphatidylinositol/phosphatidylserine/DHE (40:40:10:8:2, mol %) and the competitive binding of ergosterol with subsequent addition of the liposomes with phosphatidylcholine/phosphatidylethanolamine/phosphatidylinositol/phosphatidylserine/ergosterol (25:25:10:10:30, mol %) at 6.5 μM and 23 nM of liposomes and protein, respectively ( Supplementary Fig. 1 ). Upc2 binds DHE and ergosterol in a similar manner to that of DOPC/DHE liposomes. Ecm22, the close homologue of Upc2, also binds to free DHE in the same manner as that of Upc2 ( Fig. 1f ). 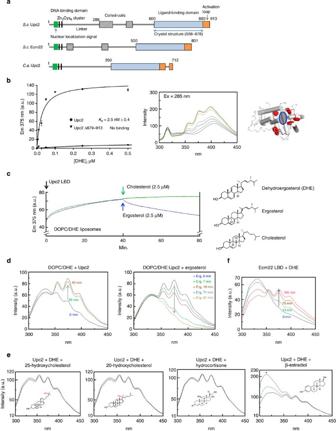Figure 1: Specific binding of Upc2 LBD to ergosterol and DHE. (a) Schematic presentation of the domain structures of Upc2 and Ecm22 inS. cerevisia(S.c.) andC. albicans(C.a.). (b) Binding curves of DHE for wild-type Upc2 LBD and the C-terminal truncation mutant of Upc2 LBD (Δ878–913). Intensities of fluorescence emission at the 375 nm of the samples (λex=285 nm) were plotted with increasing amounts of DHE concentrations. Each data point shown is the average of three measurements with error bars representing the s.d. Fit curves to data points were calculated based on one-site-binding model. One set of fluorescence emission spectra for wild-type Upc2 LBD was shown in the right panel. Five tryptophan residues that are located within 15 Å from the binding pocket were indicated by red spheres on the right panel. (c) Real-time measurement of DHE extraction by Upc2 LBD from large DOPC liposomes. The liposomes contained total 124 μM of phosphatidylcholine and DHE in a 98:2 molar ratio. Upc2 LBD was added to the liposomes with the final concentration of 0.73 μM at the beginning of kinetic measurement. Non-fluorescent ergosterol or cholesterol was added to the final concentration of 2.5 μM at 40 min for competitive binding to DHE. (d) Fluorescence emission spectra (λex=285 nm) of the samples during and at the end of the kinetics are shown forc. (e) Fluorescence emission spectra (λex=285 nm) of various sterols for competitive binding to DHE. The 0.6 μM of Upc2 LBD was loaded with 2.5 μM of free DHE. Three different lines in each experiment represent different concentrations of competing ligands (25-hydroxycholesterol, 20-hydroxycholesterol, hydrocortisone and β-estradiol) with 2.5, 4 and 10 μM respectively. β-estradiol is a naturally fluorescent compound. Asterisk indicates the intrinsic fluorescence emission of β-estradiol at 310 nm (λex=285 nm). (f) Fluorescence emission spectra of Ecm22 LBD on DHE binding. Figure 1: Specific binding of Upc2 LBD to ergosterol and DHE. ( a ) Schematic presentation of the domain structures of Upc2 and Ecm22 in S. cerevisia ( S.c. ) and C. albicans ( C.a. ). ( b ) Binding curves of DHE for wild-type Upc2 LBD and the C-terminal truncation mutant of Upc2 LBD (Δ878–913). Intensities of fluorescence emission at the 375 nm of the samples ( λ ex =285 nm) were plotted with increasing amounts of DHE concentrations. Each data point shown is the average of three measurements with error bars representing the s.d. Fit curves to data points were calculated based on one-site-binding model. One set of fluorescence emission spectra for wild-type Upc2 LBD was shown in the right panel. Five tryptophan residues that are located within 15 Å from the binding pocket were indicated by red spheres on the right panel. ( c ) Real-time measurement of DHE extraction by Upc2 LBD from large DOPC liposomes. The liposomes contained total 124 μM of phosphatidylcholine and DHE in a 98:2 molar ratio. Upc2 LBD was added to the liposomes with the final concentration of 0.73 μM at the beginning of kinetic measurement. Non-fluorescent ergosterol or cholesterol was added to the final concentration of 2.5 μM at 40 min for competitive binding to DHE. ( d ) Fluorescence emission spectra ( λ ex =285 nm) of the samples during and at the end of the kinetics are shown for c . ( e ) Fluorescence emission spectra ( λ ex =285 nm) of various sterols for competitive binding to DHE. The 0.6 μM of Upc2 LBD was loaded with 2.5 μM of free DHE. Three different lines in each experiment represent different concentrations of competing ligands (25-hydroxycholesterol, 20-hydroxycholesterol, hydrocortisone and β-estradiol) with 2.5, 4 and 10 μM respectively. β-estradiol is a naturally fluorescent compound. Asterisk indicates the intrinsic fluorescence emission of β-estradiol at 310 nm ( λ ex =285 nm). ( f ) Fluorescence emission spectra of Ecm22 LBD on DHE binding. Full size image To compare the sterol ligands identified by in vitro experiments with the natural ligand captured by Upc2 from yeast cell lysate, we characterized the ligand extracted by Upc2 using reversed-phase high-performance liquid chromatography (HPLC) and liquid chromatography-mass spectroscopy analyses ( Fig. 2 ). The captured ligand was exclusively ergosterol with no detectable species of other lipids. Given the similarities in structural and chemical properties between ergosterol and DHE, and that ergosterol is far more abundant than DHE in yeast cells, we concluded that ergosterol is a physiological ligand for Upc2. 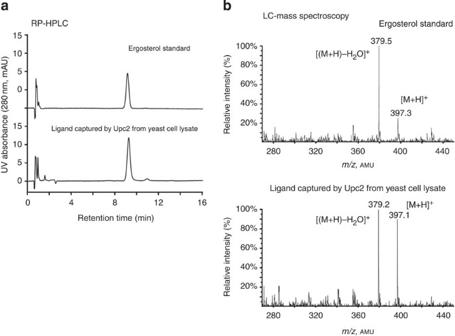Figure 2: HPLC and liquid chromatography-mass spectrometry analyses of the ligand captured by Upc2 from yeast cell lysate. (a) Reversed-phase HPLC elution profile of pure ergosterol standard (Sigma 45480) and the ligand extracted from Upc2 LBD. (b) Mass spectroscopy analysis of ergosterol standard and the ligand extracted from Upc2 LBD. Identification of the ligand captured by Upc2 was achieved by comparison of chromatographic properties and mass spectroscopy with the reference standard and literature data56.AMU, atomic mass unit; UV, ultraviolet. Figure 2: HPLC and liquid chromatography-mass spectrometry analyses of the ligand captured by Upc2 from yeast cell lysate. ( a ) Reversed-phase HPLC elution profile of pure ergosterol standard (Sigma 45480) and the ligand extracted from Upc2 LBD. ( b ) Mass spectroscopy analysis of ergosterol standard and the ligand extracted from Upc2 LBD. Identification of the ligand captured by Upc2 was achieved by comparison of chromatographic properties and mass spectroscopy with the reference standard and literature data [56] . AMU , atomic mass unit; UV, ultraviolet. Full size image Upc2 LBD displays a novel α-helical fold To examine the structure of the C-terminal LBD of Upc2, we performed the crystallographic studies on various C-terminal constructs. The crystals of apo Upc2 LBD and ergosterol-bound Upc2 LBD were crystallized but they did not diffract at synchrotron radiation. To improve the diffraction quality of Upc2 LBD crystals, we engineered a fusion protein (Upc2 LBD–T4L) in which T4 lysozyme replaces the variable loop (residues 715–725) in Upc2 (ref. 28 ). Upc2-T4L fusion protein was expressed stably and displayed good DHE-binding properties ( Fig. 3a ), which suggests that the T4 lysozyme fusion does not interfere with the ligand binding and the protein folding. The structure of the C-terminal LBD of apo Upc2 (residues 598–878)-T4L lacking the C-terminal 35 residues was determined to 2.9 Å resolution by the single anomalous dispersion method using selenomethionine-labelled crystals. The final structure containing two molecules of Upc2-T4L and 29 water molecules in the asymmetric unit was refined to an R -factor of 24.9% ( Table 1 ). 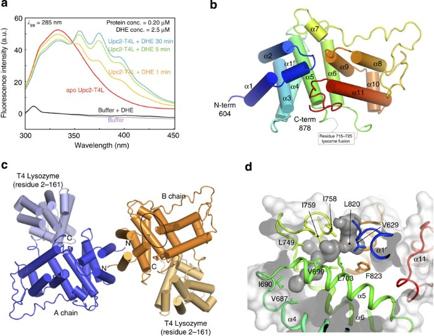Figure 3: Structure of Upc2 LBD. (a) Fluorescence emission spectra of Upc2 LBD–T4L fusion construct (residues 598–913) on DHE binding. (b) Overall structure of Upc2 LBD. The structure was coloured with red to blue based on the secondary structure succession. The T4 lysozyme fused in the α5–α6 loop was not shown for clarity. (c) Overall structure of Upc2 LBD–T4L dimer with cylindrical representation. The location of deep hydrophobic pocket in one of the Upc2 protomers is indicated by a black circle. (d) Surface representation of Upc2 LBD monomer. The residues composing the wall of the hydrophobic pocket are shown in sticks. The hydrophobic pocket is shown in grey surface representation. Conc., concentration; C-term, C-terminal; N-term, N-terminal. Figure 3: Structure of Upc2 LBD. ( a ) Fluorescence emission spectra of Upc2 LBD–T4L fusion construct (residues 598–913) on DHE binding. ( b ) Overall structure of Upc2 LBD. The structure was coloured with red to blue based on the secondary structure succession. The T4 lysozyme fused in the α5–α6 loop was not shown for clarity. ( c ) Overall structure of Upc2 LBD–T4L dimer with cylindrical representation. The location of deep hydrophobic pocket in one of the Upc2 protomers is indicated by a black circle. ( d ) Surface representation of Upc2 LBD monomer. The residues composing the wall of the hydrophobic pocket are shown in sticks. The hydrophobic pocket is shown in grey surface representation. Conc., concentration; C-term, C-terminal; N-term, N-terminal. Full size image Table 1 Data collection and refinement statistics. Full size table The structure of apo Upc2 LBD displays a globular α-helical fold with an oval shape ( Fig. 3b ). The Upc2 LBD is composed of 11 α-helices and connecting loops. There is a small predicted α-helix (α12, residues 889–896) in the C-terminal loop region that was not included in the crystallized construct. The 11 α-helices are arranged to form a closed clamp that creates a deep pocket in the core of the protein. The first three α-helices compose the N-terminal fingers and the helices α8–α9, α7 and α11 compose the other fingers of the clamp. The four helices α3–α6 compose the central palm as a helical bundle. The α7–α8 loop (residues 760–799) surround the helices α8–α9 as a longest random coil in the structure. The T4 lysozyme replacing nine residues in the α5–α6 loop is closely located on the surface of Upc2 LBD ( Fig. 3c ). The structure of Upc2 LBD reveals a central hydrophobic pocket surrounded by α helices ( Fig. 3d ). The deep hydrophobic pocket has a volume of 287 Å 3 . The helices α5 and α6 compose the bottom of the pocket and the helices α1–α2, α7, α9 and α11 compose the wall of the hydrophobic binding pocket. The pocket is accessible to a solvent with a small pore on the surface. The presence of a hydrophobic pocket suggested to us that it may serve as a binding site for small lipophilic molecules. Structural comparison of Upc2 with known structures in the PDB using the DALI server did not find related structures with Z scores >7 suggesting that the Upc2 LBD represents a novel fold of a LBD. Upc2 LBD forms a constitutive homodimer Size-exclusion chromatography (SEC) analysis demonstrated that the recombinant Upc2 LBD or Upc2 LBD–T4L is a homogeneous dimer without a detectable monomeric species, suggesting that dimeric Upc2 is a biologically relevant form. The dimer of Upc2 LBD contains two sterol-binding sites and the ligand binding did not affect the oligomeric state of Upc2 as analysed by SEC ( Fig. 4a ). There were two molecules of Upc2 LBD–T4L related by a non-crystallographic two-fold axis in the asymmetric unit of the crystals. Upc2 LBD dimerizes by helices α1 and α2 forming a four-helix bundle in the dimer interface ( Fig. 4b ). The N termini of Upc2 LBD dimer are exposed to the same side near the center of dimer interface. The dimer interface is mainly composed of hydrophobic residues burying 1,562 Å 2 of surface area at the interface ( Fig. 4c ). The Met610 is located in the center of dimer interface. M610R mutant is a monomer in solution analysed by SEC suggesting that the dimer observed in the crystal structure is consistent with that observed in solution ( Fig. 4a ). The LBDs of C. albicans Upc2 and S. cerevisiae Ecm22 are also dimers in solution and the M506R mutation of C. albicans Upc2 led to the monomerization of the LBD. The conservation of the residues composing the dimer interface in Upc2 homologues suggests that the homodimerization of LBDs is a general feature of these proteins ( Supplementary Fig. 2 ). 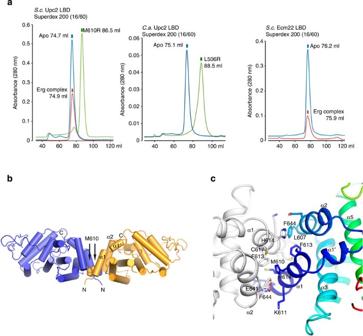Figure 4: Upc2 LBD forms a dimer. (a) Profiles of SEC for LBDs ofS. cerevisiae(S.c.) Upc2,C. albicans(C.a.) Upc2 andS. cerevisiaeEcm22. Profiles of wild type and the dimer interface mutants (M610R inS. cerevisiaeUpc2 and L506R inC. albicansUpc2) are shown in blue and green, respectively. The profiles of ergosterol-bound Upc2 and Ecm22 LBDs are shown in red lines. Ergosterol-bound LBDs were prepared by mixing purified LBDs and ergosterol in a 1:5 molar ratio and the mixture was incubated overnight before SEC analysis. (b) Side view of the Upc2 LBD dimer. (c) Detailed view of the Upc2 dimer interface. One protomer is shown in rainbow color and the other in white. Figure 4: Upc2 LBD forms a dimer. ( a ) Profiles of SEC for LBDs of S. cerevisiae ( S.c. ) Upc2, C. albicans ( C.a. ) Upc2 and S. cerevisiae Ecm22. Profiles of wild type and the dimer interface mutants (M610R in S. cerevisiae Upc2 and L506R in C. albicans Upc2) are shown in blue and green, respectively. The profiles of ergosterol-bound Upc2 and Ecm22 LBDs are shown in red lines. Ergosterol-bound LBDs were prepared by mixing purified LBDs and ergosterol in a 1:5 molar ratio and the mixture was incubated overnight before SEC analysis. ( b ) Side view of the Upc2 LBD dimer. ( c ) Detailed view of the Upc2 dimer interface. One protomer is shown in rainbow color and the other in white. Full size image The C-terminal loop is essential for ligand binding The majority of the constitutive activation mutations in S. cerevisiae Upc2 and C. albicans Upc2 are clustered in the C-terminal loop between helix α11 and the predicted α12 helix [21] , [29] . The crystal structure does not include this C-terminal activation loop of 35 residues. To examine the functional importance of this C-terminal loop, we performed the ligand-binding assays on the C-terminal deletion mutants of Upc2 LBD ( Fig. 5a ). Truncation of the C-terminal 14 residues (Δ900–913) did not affect ligand binding. However, deletion of the C-terminal 35 residues (Δ879–913), including the predicted α12, abolished DHE binding, suggesting that the C-terminal glycine rich loop and helix α12 are essential for ligand binding ( Fig. 5b ). In addition, G888D, a constitutive activation mutation in the α11–α12 loop inhibited DHE binding significantly. 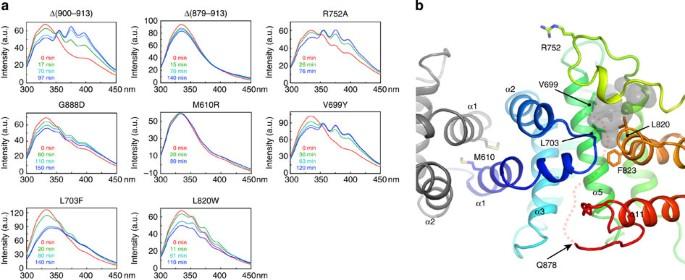Figure 5: Sterol-binding pocket of Upc2. (a) Fluorescence emission spectra of various mutants on DHE binding. The emission spectra at several time points were shown in different colours. (b) Ribbon representation of the hydrophobic pocket. The hydrophobic pocket is shown in grey surface representation. The speculative trace of the C-terminal activation loop that was not included in the crystallized construct is shown in red dots. Figure 5: Sterol-binding pocket of Upc2. ( a ) Fluorescence emission spectra of various mutants on DHE binding. The emission spectra at several time points were shown in different colours. ( b ) Ribbon representation of the hydrophobic pocket. The hydrophobic pocket is shown in grey surface representation. The speculative trace of the C-terminal activation loop that was not included in the crystallized construct is shown in red dots. Full size image The crystal structure of Upc2 LBD shows a deep hydrophobic pocket that might accommodate a single sterol molecule. However, the size of the binding pocket in apo Upc2 LBD lacking the C-terminal activation loop is slightly smaller than the dimensions of ergosterol implying that Upc2 LBD must undergo a conformational change on ligand binding. To identify the structural determinants for sterol binding of Upc2, we tried to co-crystallize Upc2 LBD with ergosterol. However, due to the poor diffraction of sterol-bound Upc2 crystals, the structural determination of the ligand complex was not possible. Alternatively, we tested the effect of several mutations in the hydrophobic pocket on sterol binding. The mutation of residues distal to the pocket, V699Y and R752A, did not affect ligand binding. Mutation of residues in the hydrophobic binding pocket to bulky residues (L703F and L820W) significantly reduced DHE binding confirming that the hydrophobic pocket accommodates sterol ( Fig. 5b ). In addition, the M610R mutation completely abolished the sterol binding, implying that the dimerization of Upc2 LBD is required for sterol binding. The LBDs of all Upc2 homologues in fungal species display a high degree of sequence conservation ( Supplementary Fig. 2 ). Specifically, the residues located in the dimerization interface, ligand-binding pocket and the C-terminal activation loop are strictly conserved. Cytosolic Upc2 relocalizes into the nucleus on activation The unique structural and ligand-binding features of Upc2 suggested to us that Upc2 may relocalize to nucleus on ligand binding in the cytosol. We examined the cellular localization of full-length Upc2 and its mutants under ergosterol-rich or ergosterol-deficient conditions. Previously, there were several conflicting reports on the localization of Upc2 in the nucleus, cytoplasm and perinuclear foci using the C-terminal green fluorescent protein (GFP) fusion [30] , [31] , [32] . However, the key determinants of Upc2 localization have not been experimentally defined. In this study, to avoid the functional interference of GFP with the C-terminal activation loop and ligand binding, GFP was tagged to the N terminus of Upc2. Wild-type Upc2 is present mostly in the cytosol with mild nuclear localization in 30% of the cell population. When the yeast cells were grown in the presence of 5 mM ergosterol, Upc2 was localized almost exclusively to the cytoplasm. However, addition of 4 μg ml −1 of fluconazole to the culture media, which inhibits the biosynthesis of ergosterol, shifted the localization of Upc2 to nucleus in an entire cell population ( Fig. 6 ). Upc2 contains a bipartite nuclear localization signal (NLS) upstream of its Zn 2 -Cys 6 cluster sequence that confers an intrinsic nuclear localization property. The deletion of NLS (residues 2–43) made Upc2 completely cytosolic. In addition, the isolated LBD (residues 598–913) or the construct lacking NLS-DBD (construct residues 283–913) was completely cytosolic regardless of sterol levels. In contrast, deletion of the C-terminal LBD (ΔLBD, construct residues 1–559) showed strong nuclear localization independent of sterol levels. These data suggest that the ergosterol-bound C-terminal LBD suppresses the nuclear transport of Upc2 by inhibiting the NLS function. The dissociation of sterol ligand from Upc2 may lead to exposure of the NLS or release Upc2 from the capture by cytosolic proteins for nuclear transport. The deletion of the C-terminal loop (Δ879–913) that disrupts ergosterol binding led to modest nuclear localization of Upc2. G888D or mutations in the sterol-binding pocket (L820W or L703F) led to strong constitutive nuclear localization of Upc2. The M610R mutation that disrupts dimerization of LBD and ligand binding shows mostly nuclear localization regardless of sterol level, suggesting that dimerization of Upc2 is essential for its regulatory function. In conclusion, these observations together with ligand-binding assays suggest that sterol binding is the key mechanism in regulating the localization of the TF. In a sterol-rich condition, Upc2 is bound to ergosterol and is present in the cytosol as a repressed form. On depletion of ergosterol, unliganded Upc2 is activated and moves to the nucleus for transcriptional activation of related genes. 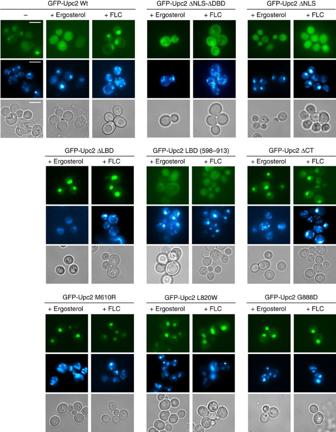Figure 6: Cellular localization of GFP-Upc2 constructs. Cells were grown in 4 μg ml−1of fluconazole or 5 mM of ergosterol for 12 h before visualization by fluorescence microscopy. Top panels show the localization of GFP-Upc2. DAPI stains both nuclear DNA as spheres and mitochondrial DNA as bright speckles which obscure features of nuclear DNA segregation. Nuclear DNA can be is distinguished from mitochondrial DNA by its size and shape. Nuclear localization of Upc2 appears as bright green spheres inside the cells. Scale bar, 3 μm. Figure 6: Cellular localization of GFP-Upc2 constructs. Cells were grown in 4 μg ml −1 of fluconazole or 5 mM of ergosterol for 12 h before visualization by fluorescence microscopy. Top panels show the localization of GFP-Upc2. DAPI stains both nuclear DNA as spheres and mitochondrial DNA as bright speckles which obscure features of nuclear DNA segregation. Nuclear DNA can be is distinguished from mitochondrial DNA by its size and shape. Nuclear localization of Upc2 appears as bright green spheres inside the cells. Scale bar, 3 μm. Full size image Upc2 regulates ergosterol level in yeast cells Upc2 and Ecm22 bind to a conserved 7-bp sterol regulatory element within promotors of most ERG genes including ERG2, ERG3 and ERG11 (refs 2 , 21 ). To investigate the mechanism of transcriptional regulation of Upc2, we check the transcriptional activity of various Upc2 constructs using ERG2 - LacZ as a reporter ( Fig. 7a ). The wild-type Upc2 displayed a moderate transcriptional activity in a normal growth condition. Fluconazole treatment increases the transcription activity more than two times. However, empty plasmid or deletion of the C-terminal LBD showed very weak transcription activity suggesting that LBD is essential for the transcriptional activity of Upc2. G888D mutation, regardless of fluconazole treatment, showed a full constitutive activation of Upc2, which is 1.2 times higher than the induced wild type. This observation is consistent with the previous report that the CTD is essential for the transcription activation of Upc2 (ref. 21 ). The M610R showed no increase of transcriptional activity on sterol depletion suggesting that dimerization is essential for the regulatory function. Deletion of the C-terminal activation loop (ΔCT) that shows constitutive nuclear localization, however, displayed at least 30% lower transcriptional activity than uninduced wild type. In addition, the transcription activity of ΔCT did not increase on fluconazole treatment. These data suggest that the C-terminal activation loop is essential not only for the regulation of protein localization but for the full transcription activity of Upc2. Disruption of sterol binding by L703F or L820W showed constitutive nuclear localization. However, the transcription activities of these mutants were 40% less than the wild type and were not enhanced significantly on fluconazole induction. It seems that introduction of bulky residues to the sterol-binding pocket not only disrupt sterol binding but also perturb the proper conformation of Upc2 for full transcriptional activity. These observations together with ligand binding and cell localization experiments suggest that sterol binding not only regulates protein localization but also regulates transcriptional activity of Upc2. To confirm that Upc2 is involved in the regulation of ergosterol level in the cells, we quantified total ergosterol contents of yeast cells containing wild-type or mutant UPC2 alleles ( Fig. 7b ). Since Upc2 activates the expression of ergosterol biosynthetic genes, it is conceivable that the sterol level of the yeast cells indirectly correlates with the transcriptional activity of Upc2. In the absence of UPC2 and ECM22 genes, sterol levels of yeast cells were weakly detectable, and the addition of 4 μg ml −1 fluconazole severely inhibited yeast cell growth. Wild-type Upc2 displayed a similar ergosterol level in the cell with those of L703F and L820W in the absence of fluconazole. The fluconazole treatment suppressed the ergosterol level by around 40% in wild type, L793F and L820W strains. Deletion of the C-terminal 35 residues (ΔCT) resulted in a slightly higher level of ergosterol than wild-type cells. However, fluconazole suppressed the sterol level of ΔCT and M610R mutant cells than wild-type cells more significantly. Upc2 lacking LBD showed some basal level of sterol synthesis in the absence of fluconazole. However, the presence of 4 μg ml −1 fluconazole inhibited the sterol level and cell growth significantly. The cells expressing G888D mutant have three times higher ergosterol levels compared with the cells expressing wild-type Upc2. Ergosterol levels were higher in fluconazole-treated G888D mutant cells compared with those found in wild-type cells grown without fluconazole. These data suggest that the G888D mutation constitutively activates Upc2 for the biosynthesis of ergosterol, which leads to an increased resistance to azole antifungals. To confirm that Upc2 is involved in the regulation of gene expression of ergosterol biosynthetic enzymes, we performed quantitative gene expression analysis of ERG11 by real-time PCR using the upc2 / ecm22 -knockout strains with wild-type and mutant UPC2 alleles. We measured the mRNA levels of ERG11 genes that were normalized by TAF10 gene as an internal control [33] . The data indicate that the mRNA expression levels of ERG11 correlate with the promotor activities of ERG2 and ergosterol levels as expected ( Supplementary Fig. 3 ). 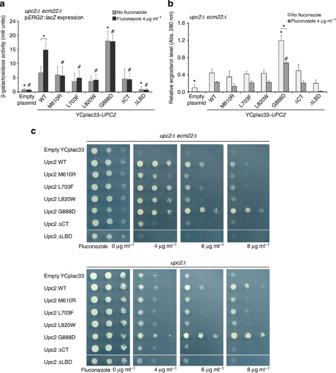Figure 7: Ergosterol level and antibiotic resistance. (a) Transcriptional activity of Upc2.ERG2-lacZreporters were used to determine the contribution of each Upc2 constructs to the regulation ofERG2promotor. β-Galactosidase assays were performed on each transformants after 5 ml cultures were grown for 16 h either in minimal medium (uninduced) or in the minimal medium containing 4 μg ml−1of fluconazole (induced). The assay values represent the average of three independent experiments. All error bars indicate s.d.Pvalues were assessed by two-tailed Student’st-test. *P<0.05 versus wild type,#P<0.05 versus each mutant without fluconazole. (b) Quantification of total ergosterol in yeast cells. Yeastupc2Δecm22Δ strains containing variousUPC2alleles were analysed for their ergosterol contents. Each data point is the average of three measurements. All error bars indicate s.d.Pvalues were assessed by two-tailed Student’st-test. *P<0.05 versus wild type,#P<0.05 versus fluconazole-treated wild-type. (c) Susceptibilities to fluconazole of yeast strains expressing wild-type or mutantUPC2allele. The strains were initially grown without fluconazole and the dilution series were spotted on the agar plates containing fluconazole and incubated for 36 h. Figure 7: Ergosterol level and antibiotic resistance. ( a ) Transcriptional activity of Upc2. ERG2-lacZ reporters were used to determine the contribution of each Upc2 constructs to the regulation of ERG2 promotor. β-Galactosidase assays were performed on each transformants after 5 ml cultures were grown for 16 h either in minimal medium (uninduced) or in the minimal medium containing 4 μg ml −1 of fluconazole (induced). The assay values represent the average of three independent experiments. All error bars indicate s.d. P values were assessed by two-tailed Student’s t -test. * P <0.05 versus wild type, # P <0.05 versus each mutant without fluconazole. ( b ) Quantification of total ergosterol in yeast cells. Yeast upc2 Δ ecm22 Δ strains containing various UPC2 alleles were analysed for their ergosterol contents. Each data point is the average of three measurements. All error bars indicate s.d. P values were assessed by two-tailed Student’s t -test. * P <0.05 versus wild type, # P <0.05 versus fluconazole-treated wild-type. ( c ) Susceptibilities to fluconazole of yeast strains expressing wild-type or mutant UPC2 allele. The strains were initially grown without fluconazole and the dilution series were spotted on the agar plates containing fluconazole and incubated for 36 h. Full size image Activation of Upc2 confers resistance to antifungal agent To investigate the relationship between the activation of Upc2 and the resistance to antifungal agents, we checked the fluconazole susceptibilities of upc2 Δ ecm22 Δ or ecm22 Δ strains expressing wild-type or mutant UPC2 alleles ( Fig. 7c ). Since fluconazole interferes with yeast cell growth by inhibiting ergosterol biosynthesis, the overall patterns of cell growths displayed a correlation with the sterol levels of the cells treated with fluconazole. Double knockout cells of upc2 Δ ecm22 Δ did not grow in the presence of fluconazole. Introduction of wild-type UPC2 permitted weak cell growth at 8 μg ml −1 of fluconazole. The yeast cells expressing a G888D mutant showed a significant increase of resistance to fluconazole at 8 μg ml −1 . However, G888D mutant grew more weakly than wild type in the absence of fluconazole suggesting that full constitutive activation of Upc2 is disadvantageous under non-selective condition by imposing metabolic burden [34] . ΔLBD mutant lacking transcription activity did not grow at the lowest fluconazole concentration. L820W, L703F, M610R and ΔCT mutants that interfere with sterol binding were more susceptible to fluconazole than the wild type. Single upc2 Δ-knockout strain harbouring ECM22 allele permitted weak growth in a low concentration of fluconazole suggesting that ECM22 has a partially overlapping role in activating genes involved in azole resistance. However, in the fluconazole concentrations higher than 6 μg ml −1 , upc2 Δ and upc2 Δ ecm22 Δ strains did not display significant differences in the susceptibilities of all Upc2 constructs, suggesting that Upc2 plays a dominant role in the sterol regulation. This is consistent with the previous observations that deletion of UPC2 results in ketoconazole sensitivity, whereas no effect was observed with ECM22 deletion suggesting that Ecm22 and Upc2 have specific targets with some essential overlapping functions [35] , [36] . Upc2 is a novel class of zinc finger TFs Recent studies proposed that several members of the fungal zinc cluster family of transcription regulators may represent functional analogues of metazoan NRs [13] , [18] , [19] , [20] . While fungal zinc cluster TFs have no apparent sequence or structural similarity to metazoan NRs, Upc2 displays conceptual similarities with steroid NRs in general domain architectures, sterol ligand binding, homodimerization, ligand-dependent transcriptional regulation and nuclear translocation. Upc2 and metazoan NRs both contain zinc finger DNA-binding domains in their N-terminal regions. Zinc fingers coordinating two zinc ions are composed of six cysteines for Upc2 and four cysteines in each of the two fingers for NRs [37] . The DNA-binding domains of NRs and zinc cluster TFs are structurally similar and they bind to DNA as homo- or heterodimers [13] . Zinc finger TFs have a C-terminal negative regulatory domain, which for a number of family members mediates ligand binding or response to small molecules such as cellular metabolites and lipophilic ligands [13] . Transcriptional activity of Upc2 is regulated by ergosterol, which is functionally similar to Type I steroid NRs in terms of ligand specificities. Upc2 and steroid receptors both form homodimers. Upc2 forms constitutive homodimers regardless of ligand binding. Oestrogen receptor α has been reported to exist as a dimer even in the apo state and the ligand binding further stabilize the homodimer [38] . Structural comparison of Upc2 with mammalian steroid NRs reveals that Upc2 has a distinctive α-helical fold of LBD from mammalian NRs ( Supplementary Fig. 4 ). Both gene regulators are mainly composed of around 12 α-helical structures with similar dimensions of LBDs. LBDs of Upc2, oestrogen and progesterone receptors form dimers by helix bundle interactions. However, except the overall configuration of dimers with ligand-binding sites closely located to the dimer interface, there is no clear structural homology between Upc2 and the NRs. On ligand binding, steroid receptors dissociate from heat shock protein Hsp90 in the cytosol and translocate to the nucleus, binding to their target gene promotors as homodimers [17] . Consistently, the translocation of Upc2 from the cytosol to the nucleus is regulated in a ligand-dependent manner. However, Upc2 LBD displays a completely different structural fold compared with the LBDs of metazoan NRs. The lack of sequence and structural similarities of fungal zinc cluster TFs and metazoan NRs suggests that the architectural and functional similarities are the product of convergent evolution with common mechanistic strategy. Phylogenetic analysis shows that the orthologues of Upc2 are only identifiable within the Saccharomycotina and Upc2/Ecm22 proteins form monophyletic clade that is not closely related to any other Zn 2 -Cys 6 proteins of Saccharomycotina [5] . The budding yeast, S. cerevisiae , contains around 50 Zn 2 -Cys 6 TFs [39] . Even though sequence homology of Upc2 to other types of zinc finger TFs is low, they harbour a conserved fungal-specific sequence within the C-terminal LBDs that was previously known as the MHR (middle homology region) [40] . The C-terminal region, including the MHR, in zinc TFs commonly contains 13–15 α-helices of secondary structure elements, which implies that the presence of a LBD is a general feature of this protein family. In conclusion, Upc2 represent a novel class of zinc finger TFs displaying a functional analogy with metazoan steroid receptors. The crystal structure of Upc2 LBD together with biochemical and yeast cell biology studies provides a detailed mechanistic picture of transcriptional regulation ( Fig. 8 ). Upc2 specifically recognizes ergosterol, which is the final product of the sterol biosynthetic pathway in fungi. Apo Upc2 localizes in the cytosol and is able to extract sterols from the lipid membranes. Since the majority of ergosterol in the cell is distributed in the plasma membranes, sensing the sterol level in the cytosol correlates well with its regulatory function. Dissociation of ergosterol leads to the relocalization of Upc2 from cytosol to nucleus. The N-terminal DNA-binding domain with NLS has an intrinsic capability of nuclear localization and the C-terminal LBD, when bound to ergosterol, masks its nuclear localization capability. Ligand-bound Upc2 might be captured by cytosolic proteins or hide the N-terminal NLS sequence from recognition by nuclear transport proteins such as importins [41] , [42] . The molecular chaperone Hsp90 mediates haem activation of the yeast zinc TF Hap1 by direct physical interactions [43] , which is similar to the mechanism of steroid NR-Hsp90 complexes in the regulation of ligand-binding, translocation and transcription [44] . The genetic interaction of Hsp90 and Upc2 in C. albicans was previously reported [45] . In addition, the Hsp90-mediated morphogenesis of C. albicans occurs via Upc2 (ref. 46 ). These studies raise interesting questions regarding the relationship of Upc2 and Hsp90 that requires further investigation. Ligand binding generally leads to transcriptional activation in many fungal Zn 6 -Cys 6 TFs [13] . Upc2 displays an inverse regulatory mechanism in which ligand binding represses the transcriptional activity of Upc2. In Upc2, the C-terminal 30 residues are defined as an ‘activation loop’. It contains a highly conserved glycine residues connected to the predicted two-turn amphipathic α-helix (α12). The activation loop in Upc2 is not only involved in sterol binding and regulation of protein localization, but also involved in transcriptional activation. The conformational flexibility of the C-terminal activation loop seems to be essential for the ligand binding and for the transcriptional regulation. Any substitution larger than alanine at G888 results in an increase of gene expression similar to that of the original G888D mutation [21] . Upc2 ΔCT does not bind DHE and it shows constitutive nuclear localization. G888D mutation in the activation loop also abolishes DHE binding, which indicate subtle changes in the activation loop have a significant influence on ligand binding properties. This suggests that the activated form of apo Upc2 LBD has a different conformation from the ligand-bound state. The structure of Upc2 LBD ΔCT shows a deep hydrophobic pocket (287 Å 3 ) that has a volume smaller than the value of ergosterol (427 Å). We suppose that the ΔCT or G888D mutations lead to an irreversible change to the activated conformation of LBD. Dissociation of ergosterol from the Upc2 LBD might result in conformational changes that liberate the C-terminal activation loop from intramolecular inhibitory contacts, allowing recruitment of transcriptional coactivators. In yeast, the mediator Gal1p/MED15 is known to play a critical role as a subunit of coactivators for Oaf1 and Pdr1 TFs [18] , [20] . Currently, the downstream coactivator of Upc2 is unknown. Discovery of the coactivator for Upc2 and the mechanistic characterization of coactivator regulation would provide important clues for the relationship between fungal zinc cluster TFs and metazoan NRs. 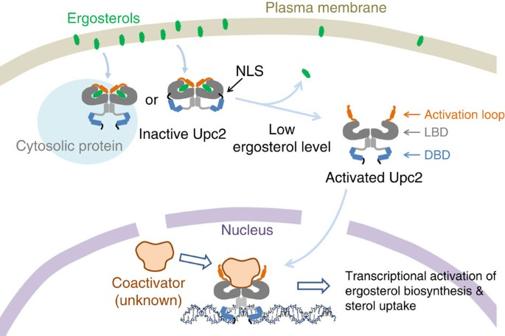Figure 8: Schematic model of transcriptional regulation by Upc2. In a sterol-rich condition, Upc2 binds to ergosterol and stays in the cytosol as a repressed form perhaps by hiding NLS or by being captured with a cytosolic protein. On ergosterol depletion, ligand-free Upc2 undergoes conformational activation and moves to nucleus for transcriptional activation of related genes. Figure 8: Schematic model of transcriptional regulation by Upc2. In a sterol-rich condition, Upc2 binds to ergosterol and stays in the cytosol as a repressed form perhaps by hiding NLS or by being captured with a cytosolic protein. On ergosterol depletion, ligand-free Upc2 undergoes conformational activation and moves to nucleus for transcriptional activation of related genes. Full size image Many zinc cluster TFs bind small-molecule intermediates, substrates or end products of the metabolic pathways that are under their transcriptional controls [13] . In contrast, many mammalian NRs bind small molecules of extracellular origin. Therefore, fungal zinc cluster TFs seem to have evolved to monitor and regulate the metabolic pathways by sensing their key compounds. Some fungal species that contains SREBP homologues do not harbour the UPC2 gene and vice versa, implying that they might have developed separate regulatory mechanism of sterol homeostasis during evolution [5] . Depletion of sterol levels by azole antifungals stimulates the activation of sterol uptake genes by Upc2 (ref. 2 ). Although there are several structural differences between cholesterol and ergosterol, they both efficiently support the growth of S. cerevisiae and C. glabrata incapable of ergosterol biosynthesis [47] . Since the human body under azole treatment provides conditions favouring the stimulation of sterol import from the fungal environment, the ability of C. glabrata to replace ergosterol with a host sterol may be responsible for its elevated azole resistance in vivo [6] , [47] . The deletion of UPC2 leads to anaerobic inviability and high susceptibility to azole antifungals in S. cerevisiae and in C. albicans [6] , [14] . Therefore, the inhibition of Upc2, which subsequently suppresses the adaptive responses of fungal cells to azoles, could be a novel strategy to improve the combined therapy with antifungal agents [16] , [48] . In this study, we uncovered the mechanism of how Upc2 senses sterol levels and activates the ergosterol biosynthetic pathway. Upc2 LBD displays a novel fold of LBD and a deep hydrophobic pocket that could serve as an excellent pharmacopore for the design of small-molecule inhibitors. In addition, Upc2 is specific to fungal sterols and has no affinities to other types of sterols providing key information for ligand-based drug design. Thus, the discovery of Upc2 as a novel class of ligand-dependent TFs opens the way for the development of new antimicrobial agents. Preparation of recombinant proteins Details of construct design, protein expression and crystallographic procedures were described elsewhere [28] . In brief, DNA encoding various portions of Upc2 (UniProt id: Q12151) was amplified by PCR using S. cerevisiae genomic DNA as a template. The PCR products were subcloned into the NdeI and XhoI sites of a pET28b vector. The variable region (residue 715–725) in Upc2 was replaced by a dipeptide sequence (Val-Asp) of the SalI restriction enzyme recognition sequence by PCR-based mutagenesis. To improve the diffraction quality of Upc2, a DNA encoding T4 lysozyme (residues 2–161) with SalI restriction enzyme sites in 5′ and 3′ overhangs was inserted into the SalI site of pET28b- UPC2 . The pET28b- UPC2-T4L (residues 598–878, 715–725Δ:: T4L ) was transferred into an Escherichia coli strain BL21(DE3) cells and the protein was expressed by addition of 0.5 mM isopropyl β- D -1-thiogalactopyranoside. Cells expressing His-Upc2-T4L were resuspended in 2 × PBS, 20 mM imidazole and were lysed by sonication. The supernatant containing His-Upc2-T4L was applied to a Ni-NTA affinity column. The eluted sample in 0.1 M Tris-HCl pH 7.5, 0.3 M imidazole, 0.3 M NaCl was concentrated to 10 mg ml −1 and the His-tag was removed by cleavage with thrombin protease. Upc2-T4L was subjected to SEC on a Superdex 200 column (GE Healthcare) equilibrated with 20 mM Tris-HCl pH 8.0, 0.3 M NaCl. The peak fractions containing Upc2-T4L were concentrated to 10 mg ml −1 for crystallization. Purification of selenomethionyl Upc2-T4L constructs essentially followed the same procedure using a methionine pathway inhibition technique using a heterotrophic E. coli strain [49] . For the ligand-binding assay, various C-terminal constructs of Upc2 and their mutants were cloned into pET28b and the proteins expressed and purified using the procedure described above. Crystallization and crystallographic analysis of Upc2-T4L Upc2 LBD–T4L crystallized in space group P3 2 with two copies in the asymmetric unit and a solvent content of 0.64. Se-SAD data sets were collected to 2.9 Å resolution at the peak wavelength of 0.97921 Å at the Photon Factory AR-NW12A beamline. SAD phasing was carried out at 3.0 Å resolution using the programme SOLVE. Twenty-two Se sites out of a total of 24 selenomethionines in the Upc-T4L dimer were found by automated heavy atom search with a figure of merit of 0.44. The phases were further improved by density modification using the programme RESOLVE [50] . The resulting electron density maps with a figure of merit of 0.70 were readily interpretable. Two molecules of Upc2 and one molecule of T4L were clearly visible in the electron density maps. The N-terminal subdomain (residues 15–56) of the second T4L molecule in the asymmetric unit was poorly defined in the electron density maps due to the disorder in the lattice. The structure of Upc2-T4L was built manually using the programme Coot [51] . The structure of Upc2-T4L was refined to R work / R free of 24.9%/27.1% using CNS [52] . The final model consisted of two copies of Upc2 (residues 604–878), two copies of T4 lysozyme (residues 2–161) and 29 water molecules. There are 95.4% of the residues in the most favoured and additional allowed regions of the Ramachandran plot. Seven residues have conformations in disallowed regions, and all of these are located in regions of high mobility at the extreme termini of chains or in the flexible loop regions. A stereo image of selected electron density is presented in Supplementary Fig. 5 . Liposomes DOPC, DOPE (1,2-dioleoyl- sn -glycero-3-phosphoethanolamine), POPS (1-palmitoyl-2-oleoyl- sn -glycero-3-phospho-L-serine), were obtained from Avanti Polar Lipids Inc. Phosphatidylinositol (soybean), ergosterol and DHE were obtained from Sigma-Aldrich. The liposomes were prepared as described with slight modifications [26] . Lipids in stock solutions in chloroform or in ethanol were mixed at the desired molar ratio, incubated at 37 °C for 5 min and the solvent was evaporated by nitrogen stream. The dried lipids were resuspended in 50 mM HEPES, pH7.2 and 120 mM potassium acetate (HK buffer) by vortexing. The liposomes were prepared at a total lipid concentration of 1.3 mM. The hydrated lipid mixture was frozen and thawed five times using water bath and cooled ethanol at −70 °C. The lipid mixture was extruded 10 times through a 0.1-μm (pore size) polycarbonate filter. Liposomes were stored at 4 °C in the dark and used within 3 days. Kinetic measurement of ligand binding using FRET Fluorescent measurements of DHE binding to Upc2 LBD were based on FRET between Trp and bound DHE and were carried out using methods as previously reported [26] , [53] . For kinetics measurements, Trp fluorescence was measured at 340 nm (bandwidth 5 nm) on excitation at 285 nm (bandwith 5 nm) in a spectrofluorometer (FP-6200; JASCO). One ml of sample initially containing the liposomes (1.3 mM) was diluted two times with HK buffer. The liposomes were diluted with the buffer to desired concentrations right before the experiments. The sample (volume 2 ml) was placed in a square quartz cell and continuously stirred with a small magnetic bar at ambient temperature. Upc2 proteins were injected into the sample cell with a final protein concentration of 0.6 μM and the kinetics measurement was started instantly. 2.5 μM of free ergosterol or cholesterol was added to the mixture at 40 min and the measurement was continued for another 40 min. Emission spectra were recorded at several time points on excitation at 285 nm. Free DHE-binding and competition assays To measure the binding affinity of Upc2 to DHE, a serial dilution series of free DHE (0, 2.5, 5, 25, 50, 100, 250 and 500 nM) were mixed with 47 nM of Upc2 LBD and incubated for 14 h. On the basis of the amounts of protein and the ligand bound, free ligand concentrations in each point were calculated and used for one-site-binding model analysis. Emission at 375 nm was recorded with maximum sensitivity of fluorometer and the binding curve was fitted with a one-site-binding model using the programme SigmaPlot. To monitor the binding of other sterol ligands, a competition assay was performed. Upc2 LBD (0.6 μM) was preloaded with DHE by incubating Upc2 and 2.5 μM of free DHE for 6 h in ice. Increasing amounts of second sterol ligands (2.5, 5.0 and 10 μM) were added and incubated for 2 h at room temperature before the emission spectra of the mixtures were recorded. Reversed-phase HPLC and MS analyses The purified His-tagged Upc2 LBD (5 mg) from E. coli in apo-form was incubated with yeast cell lysate (50 ml culture) for 30 min at room temperature. Upc2 LBD was isolated by Ni-NTA affinity chromatography. The sterol ligand captured by Upc2 was extracted to n -heptane as described [54] . Three ml of 25% alcoholic potassium hydroxide solution was added to Upc2 LBD sample and vortex mixed for 1 min and the mixture was incubated at 85 °C for 1 h. Sterols were then extracted by addition of a mixture of 1 ml of distilled water and 3 ml of n -heptane followed by vortex mixing for 3 min. The heptane layer containing extracted sterol was collected for subsequent chromatographic analysis. Heptane was vacuum dried out and the sterol pellet was solubilized in methanol. The samples dissolved in methanol were analysed by RP-HPLC (Shimadzu 10Avp HPLC system) with a Thermo Hypersil BDS (C8) 50 × 3 mm, 3 μm column and coupled with a triple-quadrupole equipped mass spectrometer (API2000, AB Sciex) with an ESI source. The mobile phase components were 0.05% trifluoroacetic acid in water and 0.05% trifluoroacetic acid in acetonitrile. We used a method based on an acetonitrile isocratic condition that allowed the detection of compounds. The products were eluted at a flow rate of 0.4 ml min −1 with 75% acetonitrile, and monitored by determining absorbance at 280 nm. Compounds were identified based on their retention times and the masses detected in the liquid chromatography-mass spectrometry system were compared with the pure ergosterol standard (Sigma 45480). Plasmid construction and yeast strains The complete expression cassette and the open reading frame of Upc2 were amplified from yeast genomic DNA and cloned into YCplac33 and pRS413MET-GFP. Mutant constructs were generated by site-directed mutagenesis and confirmed by DNA sequencing. The upc2 Δ ecm22 Δ strain was prepared by replacing the ECM22 gene with LEU2 gene from an upc2 Δ strain (BY4741, MATa his3Δ1 leu2Δ0 met15Δ0 ura3Δ0 ) by homologous recombination. Plasmids encoding the UPC2 gene were transformed to the upc2 Δ ecm22 Δ strain (BY4741, MATa his3Δ1 leu2Δ0 met15Δ0 ura3Δ0 ecm22 Δ:: LEU2 ). Fluconazole susceptibility test Fluconazole susceptibility testing was performed by introducing YCplac33 plasmids containing the full expression cassette of wild-type or mutant UPC2 into the upc2 Δ ecm22 Δ strain. The transformed cells were grown at 30 °C until the cell density reached to OD 600 of 1. The serial dilutions of cells were spotted on agar plates containing fluconazole and incubated for 36 h. Microscopy Yeast strains expressing the appropriate GFP-UPC2 alleles were grown to an OD 600 of 0.4–0.6 in selection media. Cells were grown with 4 μg ml −1 of fluconazole or 5 mM ergosterol. Yeast cells were labelled by adding DAPI (4′,6-diamidino-2-phenylindole) at a final concentration of 5 μg ml −1 for mitochondrial and nuclear DNA staining. The cells were further incubated for 1 h before harvesting. The cells were washed two times with 1 × PBS and resuspended in selection media for observation under the microscope. Visualization of cells was performed on an Eclipse Ti fluorescence microscope (Nikon) equipped with fluorescein isothiocyanate and DAPI filters and the images were captured with an Andor ixon EMCCD camera. Measurement of transcription activity pRS413- ERG2-lacZ was an ERG2-lacZ reporter made by subcloning an ERG2 promoter, lacZ DNA, into the multiple cloning sites of the pRS413MET vector. ERG2 promotor from −751 to −1 was amplified by PCR from yeast genomic DNA. lacZ was amplified by PCR from E. coli genomic DNA. The 3′ end of ERG2 promotor was fused to the 5′ end of lacZ open reading frame by PCR amplification. ERG2-lacZ DNA was subcloned to BamHI/XhoI sites of pRS413 vector. pRS413- ERG2-lacZ and the YCplac33- UPC2 construct were co-transformed to the upc2 Δ ecm22 Δ strain. Five ml of yeast cells were grown to an OD 600 of 1 and the activity of β-galactosidase was measured as described [55] . Sterol quantification of yeast cells Total intracellular sterols were extracted as described [54] with slight modifications. In brief, 5 ml overnight culture from a single S. cerevisiae colony was used to inoculate 50 ml of a selection medium containing 0, or 4 μg ml −1 of fluconazole. The cultures were incubated for 16 h at 30 °C. The stationary-phase cells were harvested by centrifugation at 2,700 r.p.m. for 5 min and washed once with distilled water. Cell densities were measured based on OD 600 of the cultures and equal amounts of cells were processed for sterol extraction. Three ml of 25% alcoholic potassium hydroxide solution (25 g of KOH and 35 ml of sterile distilled water, brought to 100 ml with 100% ethanol) was added to each pellet and vortex mixed for 1 min. Cell suspensions were transferred to glass tubes and were incubated in an 85 °C water bath for 1 h. Following incubation, the tubes were allowed to cool to room temperature. Sterols were then extracted by addition of a mixture of 1 ml of distilled water and 3 ml of n -heptane followed by vortex mixing for 3 min. The heptane layer was transferred to a clean tube and stored at −20 °C. Before analysis, a 20-μl aliquot of sterol extract was diluted fivefold in 100% ethanol and scanned spectrophotometrically between 240 and 300 nm with a NanoDrop 1000 Spectrophotometer (Thermo Fisher Scientific). The presence of ergosterol and DHE in the extracted sample resulted in a characteristic four-peak curve. Accession codes: Coordinates and structure factors for the reported crystal structure have been deposited in the Protein Data Bank with the accession code, 4N9N . How to cite this article : Yang, H. et al . Structural mechanism of ergosterol regulation by fungal sterol transcription factor Upc2. Nat. Commun. 6:6129 doi: 10.1038/ncomms7129 (2015).